NMR spectroscopic detection of chirality and enantiopurity in referenced systems without formation of diastereomers Enantiomeric excess of chiral compounds is a key parameter that determines their activity or therapeutic action. The current paradigm for rapid measurement of enantiomeric excess using NMR is based on the formation of diastereomeric complexes between the chiral analyte and a chiral resolving agent, leading to (at least) two species with no symmetry relationship. Here we report an effective method of enantiomeric excess determination using a symmetrical achiral molecule as the resolving agent, which is based on the complexation with analyte (in the fast exchange regime) without the formation of diastereomers. The use of N,N′-disubstituted oxoporphyrinogen as the resolving agent makes this novel method extremely versatile, and appropriate for various chiral analytes including carboxylic acids, esters, alcohols and protected amino acids using the same achiral molecule. The model of sensing mechanism exhibits a fundamental linear response between enantiomeric excess and the observed magnitude of induced chemical shift non-equivalence in the 1 H NMR spectra. Chirality plays a key role in many biological events but is also important in the development of new pharmaceuticals [1] , for control of organic asymmetric reactions [2] , chiral catalysis [3] , [4] and in several aspects of supramolecular science [5] , [6] , [7] , [8] , [9] , [10] . Therefore, the detection of chirality, including analysis of chiral purity and interactions between chiral species, is an intensive area of research. Various procedures for determining analyte chirality have been proposed and those of note are based on optical (for example ultraviolet/visible spectrophotometry (uv/Vis) [11] , [12] , [13] , circular dichroism (CD) [14] , [15] , fluorescence [16] , [17] , [18] , [19] ) and electrochemical [20] methods involving a synthetic chiral host as a chirality detector. However, the use of an achiral host as a detector has only seldom been achieved, that is, through the formation of ternary diastereomeric complexes between chiral substrate molecules and achiral host [21] or by the observation of exciton-coupled CD effects in porphyrin tweezer molecules where helicity is induced by complexation with a chiral guest [22] , [23] , [24] , [25] . Over several decades NMR spectroscopic methods, which depend on a chiral auxiliary such as chiral derivatization agent [26] , [27] , [28] , chiral lanthanide shift reagents [26] , [29] and chiral solvating agents (CSA) [27] , [28] , [29] , [30] have been extensively studied. NMR discrimination methods that do not use an auxiliary have also been developed [31] , [32] , [33] although they are considered unusual as self-association between chiral analytes is required in the formation of diastereomeric dimers. Use of an achiral auxiliary in conjunction with 31 P NMR spectroscopy has also been reported [34] . However, in that case an achiral derivatization agent was used as a platform for covalent coupling of two chiral analyte molecules resulting in diastereomer formation and three well-separated NMR resonances could be observed. We have previously reported a method that facilitates the latter concept by using a solvating agent where a host–guest complex (formed via non-covalent interaction) between an achiral host and two chiral guests is formed [35] , [36] . In that case, formation of two rapidly exchanging diastereomers occurs and resulting NMR spectra show two distinct resonances whose separation reflects proportionally the enantiomeric excess of the chiral guest. Chiral liquid crystals [37] , [38] , [39] have been used as anisotropic solvents to differentiate enantiotopic directions of prochiral analyte molecules without diastereomer formation although in that case the analyte resonances are observed (however, if chiral analyte molecules are dissolved in chiral liquid crystals diastereomeric pairs are formed). Based on these examples it seems that NMR, as an intrinsically achiral method, lacks the capability to sense chirality or enantiomeric excess (e.e.) in the absence of a chiral auxiliary, or of self-association of chiral analytes, or without formation of at least 1:2 complexes of achiral agent:chiral analyte. In all cases, formation of diastereomeric species occurs in solution and utilization of NMR in conjunction with an achiral reagent in non-diastereomeric binding mode as a probe of enantiopurity remains challenging. Such processes where ‘achiral’ can sense ‘chiral’ might have connotations for enantioselective amplification, as well as for the origin of homochirality in living organisms [40] . In this work, we introduce a 1 H NMR versatile prochiral solvating agent (pro-CSA) for determination of chirality and e.e. which does not rely on formation of diastereomeric pairing between prochiral host and chiral analyte; rather, a pair of enantiomeric complexes are formed. Detection of information about a chirality/e.e. without employing formation of diastereomers has not to our knowledge been reported and is an unusual and intriguing aspect of our pro-CSA host. The pro-CSA host molecule contains appropriate prochiral CH reporter groups, which facilitate e.e. discrimination. The nature of chirality detection and e.e. sensing are rationalized in terms of 1:1 host–guest complexation between pro-CSA molecule, represented by the N,N′-disubstituted oxoporphyrinogen host molecule H , and various chiral guest molecules G* , including carboxylic acids and esters, amino acid esters, N-protected amino acids, and some terpenoids such as menthol and camphor. Experimental and theoretical methods (NMR, uv/Vis, CD, quantum mechanical (QM) calculations and classical molecular dynamics (MD) simulations) are used to elucidate the chirality and/or e.e. sensing properties of the system presented here. Symmetry and origin of chemical shift non-equivalence The e.e. discrimination method presented here relies fundamentally on the concept of prochirality [41] , defined as ‘the geometric property of an achiral object (or spatial arrangement of points or atoms) which is capable of becoming chiral in a single desymmetrization step’ [42] . It is known that when a prochiral compound (for example, an achiral primary carboxylic acid Ph(CH 2 )CO 2 H) is placed in a chiral environment (for example, (+)-(1 R ,2 R )-1,2-diphenylethane-1,2-diamine) forming an acid-amine complex, the enantiotopic (prochiral) methylene hydrogens of the acid exhibit chemical shift non-equivalency and thus are rendered diastereotopic [43] , [44] . The pro-CSA, H , presented here contains enantiotopic CH reporter groups as shown in Fig. 1a . When an enantiopure chiral guest ( Fig. 1b ) is added to a solution of host molecule H symmetrical splitting (sometimes with an associated up- or downfield shift) of the resonance due to the reporter groups can be observed ( Fig. 1c ). H complexes with a chiral guest by hydrogen bonding through pyrrolic NH groups located at its centre resulting in downfield shift of the NH proton resonance ( Fig. 1c ). Taking into account the host’s saddle shape and the relative rigidity of its macrocycle, the distance of the available CH reporter groups from the binding site has an important role. Each CH group exhibits different sensitivity (that is, magnitude of non-equivalency) to different chiral guests ( Fig. 1c ). As H has four such groups of practical use at different spatial positions (accessibility) and distances from the binding site there is a good chance that any chiral guest with affinity to bind to H will cause non-equivalency in selected or all of the CH reporter groups. 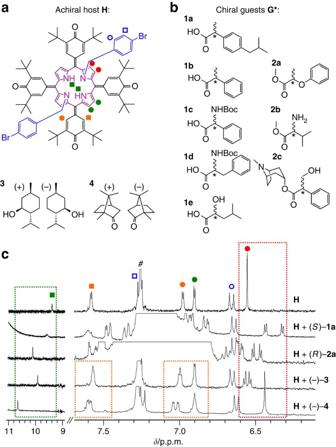Figure 1: Structures of host and guests and their NMR properties. (a) Structure of achiral host N21,N23-bis(4-bromobenzyl)-5,10,15,20-tetrakis(3,5-di-t-butyl-4-oxocyclohexadien-2,5-ylidene)porphyrinogen,H. Symbols denote the peak assignments in all1H NMR spectra in this study. (b) Structure of chiral guests used: ibuprofen1a, 2-phenylpropionic acid1b, N-boc-2-phenylglycine1c, N-boc-phenylalanine1d, leucic acid1e, 2-phenoxypropionic acid methyl ester2a, valine methyl ester2b, atropine (hyoscyamine)2c, menthol3and camphor4(boc=tert-butoxycarbonyl). (c) Typical1H NMR spectra of chloroform-dsolution of neatH(ca. 0.7 mM) andH(ca. 0.7 mM) with ca. 400 equiv. of selected chiral guests. Key: Green square (pyrrolic NH); enantiotopic CH reporter groups: orange square and circle (hemiquinonoidortho-H), green circle (N-H pyrrolic β-H) and red circle (N-alkylated pyrrolic β-H). Hash symbol denotes residual chloroform (CHCl3). FullHspectrum assignment is provided inSupplementary Figs S1–S3. Figure 1: Structures of host and guests and their NMR properties. ( a ) Structure of achiral host N 21 ,N 23 - bis (4-bromobenzyl)-5,10,15,20- tetrakis (3,5-di- t -butyl-4-oxocyclohexadien-2,5-ylidene)porphyrinogen, H . Symbols denote the peak assignments in all 1 H NMR spectra in this study. ( b ) Structure of chiral guests used: ibuprofen 1a , 2-phenylpropionic acid 1b , N-boc-2-phenylglycine 1c , N-boc-phenylalanine 1d , leucic acid 1e , 2-phenoxypropionic acid methyl ester 2a , valine methyl ester 2b , atropine (hyoscyamine) 2c , menthol 3 and camphor 4 (boc= tert -butoxycarbonyl). ( c ) Typical 1 H NMR spectra of chloroform- d solution of neat H (ca. 0.7 mM) and H (ca. 0.7 mM) with ca. 400 equiv. of selected chiral guests. Key: Green square (pyrrolic NH); enantiotopic CH reporter groups: orange square and circle (hemiquinonoid ortho -H), green circle (N-H pyrrolic β-H) and red circle (N-alkylated pyrrolic β-H). Hash symbol denotes residual chloroform (CHCl 3 ). Full H spectrum assignment is provided in Supplementary Figs S1–S3 . Full size image At this point, the origin of chemical shift non-equivalency of CH reporter groups can be elucidated in terms of the symmetry of H and disruption thereof upon interaction with a chiral guest. The term ‘prochirality’ is frequently used to describe systems where replacement of a single ligand leads to a stereogenic centre [45] . The equivalent of this in non-covalently interacting systems would be the formation of diastereotopic nuclei from initially enantiotopic nuclei due to an external factor as illustrated above in the case of acid-amine complexes where the methylene carbon of Ph(CH 2 )CO 2 H can be considered a ‘stereogenic centre’. However, the CH reporter groups of H do not posses the property that any of its carbon atoms could be converted to a ‘stereogenic centre’. For simplicity let us consider the complexation of H with 1a where the CH reporter groups of interest are at the β positions of the N-alkylated pyrrole group (β-H; Fig. 2a ). In the structure of H , two prochiral planes [44] are present ( Fig. 2a ). More specifically, two onefold improper rotations S 1 (=mirror planes σ d ), which are identical with prochiral planes, can be identified. These mirror planes make group A and B of β-H interconvertible and hence enantiotopic (magnetically equivalent with isochronous NMR resonances) [44] , [46] . 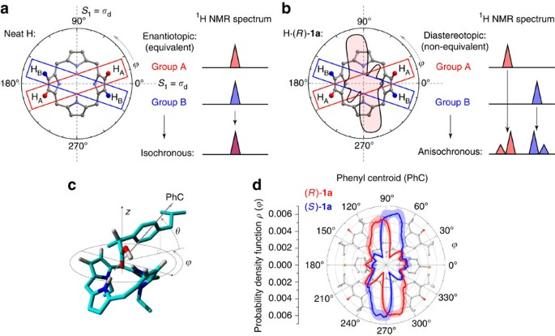Figure 2: Effect of guest complexation on symmetry of the host molecule. (a) Scheme of symmetry of host molecule and corresponding shape of NMR spectra. Dashed lines denote axes ofS1symmetry elements (mirror planes) also identical to prochiral planes. (b) Disruption of host’s symmetry upon complexation with chiral guest and resulting splitting of NMR spectral pattern. (c) Schematic plot of reference system connected with host and orientation of guest within it usingφandθcoordinates used in the MD simulations. (d) Plot of probability density functionρ(φ) as obtained from MD simulations (forH·(R)–1aandH·(S)–1acomplexes) for phenyl centroid (PhC). Solid red or blue lines show averageρ(φ) over 5°. Light red or blue background denotes standard variance ofρ(φ).Supplementary Movie 1depicts MD of the spontaneous release of (S)-1afrom the binding site with subsequent binding of (R)-1a(video length in real time is 4.4 ns). Figure 2: Effect of guest complexation on symmetry of the host molecule. ( a ) Scheme of symmetry of host molecule and corresponding shape of NMR spectra. Dashed lines denote axes of S 1 symmetry elements (mirror planes) also identical to prochiral planes. ( b ) Disruption of host’s symmetry upon complexation with chiral guest and resulting splitting of NMR spectral pattern. ( c ) Schematic plot of reference system connected with host and orientation of guest within it using φ and θ coordinates used in the MD simulations. ( d ) Plot of probability density function ρ ( φ ) as obtained from MD simulations (for H ·( R )– 1a and H ·( S )– 1a complexes) for phenyl centroid (PhC). Solid red or blue lines show average ρ ( φ ) over 5°. Light red or blue background denotes standard variance of ρ ( φ ). Supplementary Movie 1 depicts MD of the spontaneous release of ( S )- 1a from the binding site with subsequent binding of ( R )- 1a (video length in real time is 4.4 ns). Full size image Note that H also possesses a proper symmetry axis C 2 , which might suggest that groups A and B are homotopic hence isochronous even in a chiral environment. However, groups A and B (as defined in Fig. 2a ) cannot be interconverted using C 2 . Therefore, in general, β-H nuclei are required to be identified as groups A and B so that they are interconvertible by improper rotation S n (including plane σ or centre of symmetry i ) and not by operation of proper symmetry axes C n [44] . In that case, groups A and B are enantiotopic. The presence of a chiral guest leads to magnetic non-equivalence of group A and B as it affects each group of protons in a different manner as can be illustrated (from MD simulations) by the preference of certain orientations of guest occupation (that is, conformations) over others as shown in Fig. 2c . A chiral environment breaks mirror symmetry and the initially enantiotopic groups A and B become diastereotopic with distinguishable anisochronous NMR resonances ( Fig. 2b ). Note that group A and B are contained in the same molecule so that no actual diastereomers are present. This is also the reason why at any arbitrary e.e. the split peaks have the identical intensities. The second-order quartet (which exhibits roofing) appears as a consequence of the close structural connection between H A and H B protons, which have a vicinal scalar 3 J -coupling constant. From QM calculations it can be identified which group of protons will experience upfield or downfield shifts (see Supplementary Fig. S4 ). QM results for the H ·( R )- 1a complex reveal that group A is shifted relatively upfield compared with group B and vice versa due to symmetry of the complex H ·( S )– 1a . NMR spectral properties and binding model Hydrogen bonding between H and chiral guest appears to be weak so that a relatively high concentration of chiral guest is required to obtain well-resolved spectral lines ( Fig. 1c ). Interestingly, if the concentration of chiral guest is kept constant and e.e. is varied then the magnitude of splitting Δ δ of spectral lines varies linearly with e.e. ( Fig. 3a–d , for other guests see Supplementary Figs S5–S14 ). The linear dependence of Δ δ on e.e. is a fundamental property of pro-CSA molecules as will be shown later. When determining the true resonance frequency of the N-alkylated pyrrolic β-H, N-H pyrrolic β-H and hemiquinonoid ortho -H spin systems it must be taken into consideration that these spins are second-order strongly coupled systems, and the fitting procedure should be carried out with appropriate care (see 1 H NMR spectra fitting in Supplementary Methods ). The characteristic roofed shape of the split N-alkylated pyrrolic β-H resonances and the cross-peaks between them in 1 H– 1 H COSY spectrum ( Fig. 3e ) clearly indicates that both peaks originate from the same host molecule. Similar cross-peaks were observed in N-H pyrrolic β-H and hemiquinonoid ortho -H in, for example, H ·(–)− 4 complex (see 1 H NMR spectra fitting in Supplementary Methods ). As e.e. tends towards 0% (that is, racemic mixture), a single set of sharp well-resolved resonances remain. At 0% e.e. 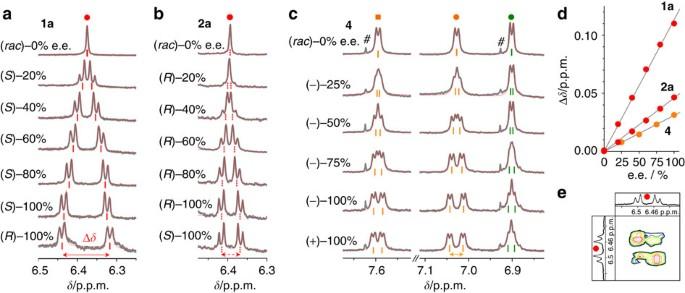Figure 3:1H NMR data showing dependency of chemical shift non-equivalency on e.e. (a,b,c) Spectra ofH(0.68 mM, chloroform-d) in the presence of various e.e. of1a(460 equiv.),2a(370 equiv.) and4(490 equiv.) at 25 °C, respectively. Hash symbol denotes carbon-13 satellite from chloroform-dsolvent. All spectra were fitted (grey=original spectrum, red=fit) and true resonance frequencies as obtained by fit are indicated by lines under each spectrum. Spectra for1aand2awere taken as AB second-order strongly coupled quartet. Left part of spectrum (orange circle and square) for guest4was fitted as two independent EF and E′F′ second-order spin systems and right part of spectrum (green circle) as CDX strongly coupled quartet of doublets (for details see1H NMR spectra fitting inSupplementary Methods). (d) Plot of dependency of Δδon the e.e. value of host’s splitted resonance (denoted by arrows ina–c) showing linear relationship (for allR2>0.997). (e) Homonuclear1H–1H COSY spectrum of N-alkylated pyrrolic β-H resonances ofH(1.42 mM, chloroform-d) with (S)-1a(200 equiv.) at 25 °C. these converge to a centred singlet for H · 1a , H · 2a and a doublet for H · 4 ( Fig 3a–c ). The lack (at 0% e.e.) of two sets of peaks, corresponding to stable complexes of H ·( R )-enantiomer and H ·( S )-enantiomer, indicates fast exchange of chiral guests at the host’s binding site. Figure 3: 1 H NMR data showing dependency of chemical shift non-equivalency on e.e. ( a , b , c ) Spectra of H (0.68 mM, chloroform- d ) in the presence of various e.e. of 1a (460 equiv. ), 2a (370 equiv.) and 4 (490 equiv.) at 25 °C, respectively. Hash symbol denotes carbon-13 satellite from chloroform- d solvent. All spectra were fitted (grey=original spectrum, red=fit) and true resonance frequencies as obtained by fit are indicated by lines under each spectrum. Spectra for 1a and 2a were taken as AB second-order strongly coupled quartet. Left part of spectrum (orange circle and square) for guest 4 was fitted as two independent EF and E′F′ second-order spin systems and right part of spectrum (green circle) as CDX strongly coupled quartet of doublets (for details see 1 H NMR spectra fitting in Supplementary Methods ). ( d ) Plot of dependency of Δ δ on the e.e. value of host’s splitted resonance (denoted by arrows in a – c ) showing linear relationship (for all R 2 >0.997). ( e ) Homonuclear 1 H– 1 H COSY spectrum of N-alkylated pyrrolic β-H resonances of H (1.42 mM, chloroform- d ) with ( S )- 1a (200 equiv.) at 25 °C. Full size image The above-mentioned features helped us to elucidate the origin of the linear relationship between magnitude of splitting Δ δ and e.e., as well as a model of the host–guest binding mechanism. The mechanism of binding should be considered as competitive involving binding of water molecules W and the chiral guest G* to the host molecule H , as titration of a chloroform solution of H with W yields a not insignificant response (and high binding constant) to traces of water ( Fig. 4a , for 1 H NMR spectra see Supplementary Fig. S15 ) [47] . Moreover, water is ubiquitous and is difficult to remove from chloroform, which also explains why a relatively high concentration of G* is required to obtain well-resolved split NMR spectra. Some examples of titrations of H with 3 are shown in Fig. 4b–e (for other guests and other types of titrations see Supplementary Figs S16–S25 ). For the two types of titration shown it can be observed that the chemical shift of pyrrolic NH resonance ( δ NH ) increases monotonically while splitting of N-substituted pyrrolic β-H (Δ δ ) does not necessarily increase monotonically (compare Fig. 4b ). These observations suggest that the NH group reflects only the overall binding of guests ( G* or W ) while the pyrrolic β-H protons are sensitive not only to overall binding but also to the nature of chiral guest and its e.e. Therefore, binding isotherms are required to be constructed (and fitted) simultaneously for both δ NH and Δ δ , as they each partially express the same characteristic (binding strength). 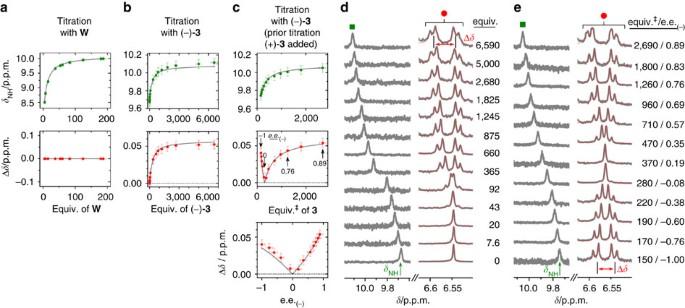Figure 4:1H NMR titration experiments supporting the competitive binding model. (a) Titration ofH(0.41 mM, chloroform-d) with waterWat 25 °C. (b) Titration ofH(0.65 mM, chloroform-d) with (–)−3at 25 °C. (c) Titration ofH(0.74 mM, chloroform-d) with (–)−3at 25 °C. Before titration (with (–)−3) 150 equiv. of (+)−3was added to the solution. Bottom panel shows dependency of Δδon e.e. during the titration. Grey curves were fitted according to a competitive binding model (seeFig. 5) using isotherms expressed in equations 2 and 3. During titrations chiral guest and water concentrations were evaluated although water concentration did not vary significantly from initial value during titration. For binding constants and other parameters seeTable 1. (d,e) Spectra taken during titration shown inb,c, respectively (grey=original spectrum, red=fit). Double dagger (‡) inc,edenotes combined concentration (in equiv.) of both enantiomers. Figure 4: 1 H NMR titration experiments supporting the competitive binding model. ( a ) Titration of H (0.41 mM, chloroform- d ) with water W at 25 °C. ( b ) Titration of H (0.65 mM, chloroform- d ) with (–)− 3 at 25 °C. ( c ) Titration of H (0.74 mM, chloroform- d ) with (–)− 3 at 25 °C. Before titration (with (–)− 3 ) 150 equiv. of (+)− 3 was added to the solution. Bottom panel shows dependency of Δ δ on e.e. during the titration. Grey curves were fitted according to a competitive binding model (see Fig. 5 ) using isotherms expressed in equations 2 and 3. During titrations chiral guest and water concentrations were evaluated although water concentration did not vary significantly from initial value during titration. For binding constants and other parameters see Table 1 . ( d , e ) Spectra taken during titration shown in b , c , respectively (grey=original spectrum, red=fit). Double dagger (‡) in c , e denotes combined concentration (in equiv.) of both enantiomers. Full size image Binding isotherms for δ NH and Δ δ can be constructed based on a 1:1 host:ligand (where ligand can be chiral guest G* or water W ) competitive binding model ( Fig. 5a ) as described by the equilibrium equations 1. 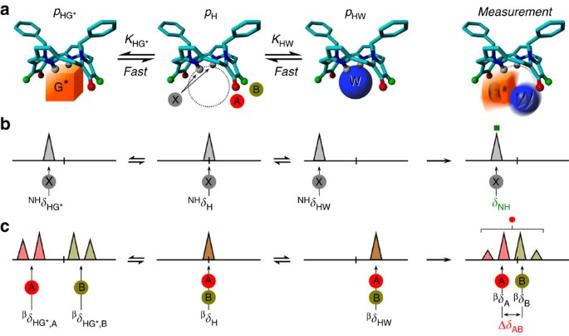Figure 5: Competitive binding model and its schematic1H NMR spectral manifestation. (a) Partial (meso-substituents removed) structural model of host,H, showing its three forms and (at right) an image illustrating the situation in solution. Equilibrium binding constants and populations are indicated. Protons of special interest (HA, HBand HX) are also highlighted. (b) Schematic description of pyrrolic NH resonance (HX) behaviour. (c) Schematic description of N-alkylated pyrrolic β-H resonances (HAand HB). Arrows indicate the true resonance frequency of spectral patterns. Figure 5: Competitive binding model and its schematic 1 H NMR spectral manifestation. ( a ) Partial ( meso -substituents removed) structural model of host, H , showing its three forms and (at right) an image illustrating the situation in solution. Equilibrium binding constants and populations are indicated. Protons of special interest (H A , H B and H X ) are also highlighted. ( b ) Schematic description of pyrrolic NH resonance (H X ) behaviour. ( c ) Schematic description of N-alkylated pyrrolic β-H resonances (H A and H B ). Arrows indicate the true resonance frequency of spectral patterns. Full size image where K HG* and K HW are the equilibrium binding constants of formation of H·G* and H·W complexes, respectively. In the derivation of binding isotherms we assume fast exchange between the three states of host H·G* , H and H·W ( Fig. 5a ) and that binding of ( R )- or ( S )-enantiomer to the host is statistical due to the symmetry of H . Then δ NH and Δ δ can be expressed in the form of equations 2 and 3 respectively (for the full derivation see Methods ). where p HG* , p HW and p H (as defined by equation 5 in Methods) are populations of all the host forms, H bound to G* or W and free H , respectively. Simultaneous fitting of the binding isotherms, δ NH and Δ δ , with experimental data yields characteristic values, in particular K HG* , Δ δ max and NH δ HG* ( Table 1 ), for each pair of host and chiral guest. These values reveal that Δ δ max is independent of K HG* and seems to be strongly related to the dynamic structural conformation of each host–guest pair. The value of Δ δ max (or Δ δ at particular concentration) for different chiral guests is, in general, not predictable (only rough estimations using density functional theory can be obtained) and without having a sample of pure enantiomer of analyte (or its known e.e. form) in hand it cannot be determined. Thus, construction of a linear calibration curve as seen in Fig. 3d seems to be a limiting factor for all pro-CSA. Table 1 Characteristic values for binding constants and isotherms. Full size table The case of the H ·( R )– 1a complex was examined in detail using density functional theory (DFT) methods. Three possible conformations of host–guest complexes ( Supplementary Data 1–3 ) and chemical shifts of N-alkylated pyrrolic β-H (for predicted value of Δ δ max see Table 1 ) were calculated (see Supplementary Fig. S4 ). From data contained in Table 1 it can be seen that all the chiral guests studied have a low equilibrium binding constant so that direct confirmation of 1:1 binding stoichiometry using Job’s plot is not feasible [48] as variation in δ NH and Δ δ was virtually unobservable when construction of a Job’s plot was attempted. However, a competitive 1:1 binding model is supported by the fact that all titration experiments for various chiral guests, QM calculations and MD simulations show good agreement with the suggested model. Equation 3 has some interesting consequences. It indicates a linear dependence on e.e., as well as on population of the H · G* complex. The apparent universal linearity of the Δ δ /e.e. plots indicates in turn that a calibration curve can always be constructed from a single measured point obtained from a sample of enantiopure analyte or a sample of independently measured e.e. (considering that a second point required for construction of a calibration curve has zero chemical shift non-equivalence Δ δ =0 for the racemate where e.e.=0). Also, the value of Δ δ can be obtained by measurement only as a non-negative value, hence, only the absolute value of e.e. can be determined and enantiomeric identity remains unknown (for example, measurement gives e.e.=80% but the excess enantiomeric form is not known). This principal indistinguishableness originates from the symmetry between enantiomeric complexes H ·( R )- G* and H ·( S )- G* and is present for all pro-CSA. It can be overcome only when a small amount of known enantiomer of guest is added. Δ δ is either increased when the same enantiomer (as that in excess in solution) is added or decreased when the other enantiomer is added [36] (an example can be seen in Fig. 4b compared with Fig. 4c ). In order to investigate the transfer of chiral information from guest to host molecule the uv/Vis and CD spectra were recorded for most of the H · G* pairs ( Supplementary Figs S26–S32 ). However, CD signal induced in the structure of H upon binding of G* is very weak (compared with other systems for example, Mizuno et al . [14] ) and can be detected only when large quantities of G* are added to solution. This is due to the rigidity of the host’s macrocyclic structure. Temperature effects on the efficiency of e.e. sensing were explored using variable temperature (VT) 1 H NMR measurements ( Supplementary Fig. S33 ). It can be seen that chemical shift non-equivalency Δ δ is decreasing with decreasing temperature. This behaviour is rather unusual since the opposite (increasing chemical shift non-equivalency) should be observed with decreasing temperature. However, this is a consequence of the competitive binding model where at depressed temperature water binds to the host more strongly than the chiral guest leading to a decrease of overall Δ δ value (which is reflected in equation 3 as a decrease of population of H · G* complex p HG* ). VT- 1 H NMR measurements also show that ambient temperature is optimal for e.e. analysis as it gives Δ δ close to the maximum values, which is practical from the point-of-view of applications. Conventional CSA and the pro-CSA sensing method presented here have different characteristics. When a conventional diastereomer-forming reagent, for example a CSA, is used two separate resonances for each enantiomer appear although they cannot be unambiguously assigned to a particular enantiomer. Additional molecular modelling or chiroptical methods (for example, CD) are required to assign enantiomer identity. However, the value of e.e. can be obtained by integration of separate resonances without having an authentic sample of analyte in advance. The non-diastereomeric sensing mechanism of pro-CSA differs conceptually from but is complementary to the existing conventional methods. From the point of practicality and potential use, the pro-CSA H presented here offers some noteworthy properties. First, when e.e. of the same analyte is required to be determined repetitively (for example, as in chemicals or pharmaceuticals industries) a calibration curve using pure enantiomers can be constructed once, which facilitates subsequent rapid analyses of e.e. by using a simple protocol. In this way, particular host–guest pairs would possess characteristic values of Δ δ under the specified conditions. This method is then also appropriate for use in various enantioenrichment (Soai reaction [49] ) studies as a rapid probe of e.e. values. In fact, in any case where initial purification (by chiral high-performance liquid chromatography or crystallization) of a chiral analyte is required (perhaps for regulatory purposes) our method should be applicable. It is also possible to perform in situ NMR monitoring of variation of e.e. without using a chiral probe, as a chiral probe might bias the outcome of, for instance, enantiomer enrichment processes [50] , [51] , [52] . Additionally, when a particular analyte is examined using conventional CSA, there exist a set of CSA suitable for each type of analyte (for example, analyte-CSA: carboxylic acids—chiral amines, aminoalcohols—carboxylic acids). Pro-CSA H based on N,N′-disubstituted oxoporphyrinogen is very versatile in this respect as it provides reasonable chemical shift non-equivalence for a great variety of analytes of different functionality. Another significant feature is that chiral information is first translated from analyte to H and then read out from H (in contrast to conventional CSAs) and, as H operates by hydrogen bonding of the analyte, it can be used to analyse many differently functionalized compounds. As a result of this, H has four sets of CH reporter groups, which can be varied synthetically (for example, to C-F groups) so that chiral information can be retrieved from 19 F NMR spectra where other resonances due to analyte and solvent are absent. Finally, this system is also of note from the point-of-view that it does not rely on the formation of diastereomers. This is perhaps counterintuitive given the prevailing opinion that formation of diastereomers is required in the analysis of e.e. In summary, a symmetrical a-/prochiral macrocyclic N,N′-disubstituted oxoporphyrinogen host molecule can be utilized as a detector of enantiomeric purity for a wide variety of guest molecules. We have shown that no diastereomeric species are present in solution as complexes with each enantiomer have identical properties. The mechanism of chiral sensing can be rationalized in terms of the host’s symmetry and its breakdown when individual host molecule interacts with chiral guest under a fast exchange regime. Chirality sensing (that is, identification of the major enantiomorph) can be achieved by addition of a portion of known enantiomer guest. When a symmetrical molecule is adapted as an e.e. sensor it has certain intrinsic advantages such as identical binding constants for each enantiomer resulting in e.e. determination, which is not obscured by kinetic resolution. The results presented here indicate that other symmetrical molecules should also be available as detectors of enantiopurity using NMR spectroscopy. Such systems might also improve our understanding of important chirality principles such as majority rule, chirality transfer between molecules and asymmetric reactions. Materials Chloroform- d (Cambridge Isotope Ltd.) for 1 H NMR spectroscopy was mostly used as received. In some specific titrations residual water was removed using 4 Å molecular sieves (Wako Chem. Co.). Before use molecular sieves were activated at 200 °C in vacuum. ( R )-ibuprofen (Nacalai Tesque), (S)-ibuprofen (TCI Co. Ltd.), ( rac )-ibuprofen (TCI Co. Ltd.), ( R )-2-phenylpropionic acid (Wako Chem. Co.), ( rac )-2-phenylpropionic acid (TCI Co. Ltd.), N-boc- L -2-phenylglycine (TCI Co. Ltd.), N-boc- D -2-phenylglycine (TCI Co. Ltd.), N-boc- L -phenylalanine (TCI Co. Ltd.), N-boc- D -phenylalanine (TCI Co. Ltd.), L -leucic acid (TCI Co. Ltd.), DL -leucic acid (TCI Co. Ltd.), (–)-hyoscyamine (TCI Co. Ltd.), (±)-hyoscyamine (TCI Co. Ltd.), (+)-menthol (Sigma-Aldrich Co. LLC. ), (–)-menthol (Wako Chem. Co.), (+)-camphor (TCI Co. Ltd.), (–)-camphor (Wako Chem. Co.) were used as received. Synthesis ( R )-2-phenoxypropionic acid methyl ester and ( S )-2-phenoxypropionic acid methyl ester were synthesized from ( R )-2-phenoxypropionic acid and ( S )-2-phenoxypropionic acid (both Wako Chem. Co.), respectively, through esterification of the corresponding carboxylic acids. 2-Phenoxypropionic acid (1.0 g), iodomethane (5 equiv.) and potassium carbonate (10 equiv.) were stirred in refluxing acetone (100 ml) for 2 h then acetone was removed under reduced pressure. Crude product was passed through a silica gel column (eluent: dichloromethane, DCM) to yield the final product as a colourless liquid. D -valine methyl ester and L -valine methyl ester were synthesized from D -valine methyl ester hydrochloride and L -valine methyl ester hydrochloride (both TCI Co. Ltd.), respectively, through neutralization of the corresponding hydrochloride salts. The hydrochloride salt was dissolved in pure water and neutralized using an excess of potassium carbonate solution (pH=c.a. 12) then the aqueous solution was extracted three times using DCM. DCM fractions were combined then dried over anhydrous sodium sulphate. Subsequent filtration and removal of DCM under reduced pressure yielded the final product as a white solid. Synthesis of host molecule N 21 ,N 23 - bis (4-bromobenzyl)-5,10,15,20- tetrakis (3,5-di- t -butyl-4-oxocyclohexadien-2,5-ylidene)porphyrinogen ( H ) has been reported previously [53] , [54] . General spectroscopic methods 1 H NMR spectra were obtained at 25 °C (unless stated otherwise) using an AL300BX spectrometer (JEOL) operating at 300.4 MHz. When variable temperature measurements (VT- 1 H NMR) were performed the appropriate JEOL temperature control unit (temperature fluctuation±0.3 °C) was used. Before the experiment, host H was dissolved in chloroform- d (usually ca. 0.6 mM) in an NMR tube and subsequently ligand (chiral guest or water) was added/injected directly into the NMR tube. Molar ratio of ligand and host was carefully determined by integration of the corresponding peaks in spectra. All spectra were referenced to tetramethylsilane. Numbers of scans typically used (for ca. 0.6 mM of host molecule H ): 16–32 scans for samples up to 500 equiv. of guest G *; 32–128 scans for samples containing from 500–1,000 equiv. of G *; 128–512 scans for samples containing in excess of 1,000 equiv. G *. Electronic absorption spectra and CD spectra were measured using a J-820 CD spectrophotometer (JASCO) at room temperature (ca. 25 °C). When titration experiments were performed a chloroform- d solution of host H (ca. 7 × 10 −5 M) was prepared and 0.17 ml of this solution was placed in a 1-mm pathlength quartz cell. In order to maintain host concentration constant chloroform- d stock solutions of host H with various chiral guests were prepared ([ H ] t ca. 7 × 10 −5 M, [ G* ] t up to ca. 1.5 M, subscript ‘t’ denotes total concentration) and subsequently titrated into the host solution by using a syringe (0–600 μl). Then uv/Vis and CD spectra were recorded simultaneously. Derivation of competitive binding model From equilibrium equations 1, the equilibrium binding constants and mass balance equations can then be expressed as equations 4. where [H] t , [G*] t and [W] t denote total concentrations of H , G* and W , respectively. [H], [G*] and [W] denote concentrations of free H , G* and W , respectively. [HG*] and [HW] are concentrations of the corresponding complexed forms. A solution (especially values of [HG*], [H] and [HW]) can be obtained using either numerical Newton iterative methods or rather complex but exact analytic solution (see Supplementary Methods ). Then populations of all the host forms (one free and two bound) can be expressed in the form of equations 5. Because of fast exchange between the three states of host H·G* , H and H·W ( Fig. 5a ) the resulting chemical shift of pyrrolic NH, δ NH , takes the form of a population averaged chemical shift of the respective states ( Fig. 5b ) and can be expressed as equation 2. Similarly, a Δ δ binding isotherm (describing chemical shift non-equivalence) can be constructed under the following assumptions. For reasons of symmetry, we assume that the binding of ( R )- or ( S )-enantiomers to the host is statistical. When a chiral guest G * binds to the host the probability that the site is occupied by ( R )- or ( S )-enantiomer can be determined as a function of e.e. by equations 6. where [G R ] t and [G S ] t are total concentrations of ( R )- and ( S )-enantiomer, respectively. As mentioned above, the 1 H– 1 H COSY spectrum of the pyrrolic β-H resonance indicates that both split peaks must be at the same pyrrolic ring. Moreover, mirror symmetry of the host’s binding site and the intrinsic saddle shape of the host’s macrocycle causes a preference for certain mutual host–guest conformations (see MD study, Fig. 2c ) and therefore does not permit isotropic rotation of guest at the binding site. Thus, when chiral guest is present, an asymmetric shielding effect at (for example) pyrrolic β-H positions occurs. In this situation, the chemical shift of respective pyrrolic β-H is given by equations 7. where β δ HG*,A and β δ HG*,B are chemical shifts of protons H A and H B (for labels see Fig. 5 ), respectively, when only chiral guests under fast exchange are considered to bind to the host molecule ( Fig. 5c ). β δ A, R and β δ A, S are chemical shifts of H A resulting from complexation with neat ( R )- and ( S )-enantiomers, respectively. β δ B, R and β δ B, S represent the same quantity for H B . β δ A, R , β δ A, S , β δ B, R and β δ B, S are constants for each specific combination of host and chiral guest (at given temperature). Symmetry and chemical shift equivalency between complexes with only ( R )- or only ( S )-enantiomer implies that β δ A, R = β δ B, S and β δ A, S = β δ B, R . For convenience let us introduce Δ δ max = β δ A, R − β δ B, R as a measure of the maximum chemical shift difference between H A and H B protons as a characteristic value for each host–guest combination. When the competitive exchange of G* with water W is taken into account the overall chemical shift β δ A and β δ B of protons H A and H B , respectively, will be described as population weighted chemical shifts ( Fig. 5c ) of respective types of host by equations 8. where β δ H and β δ HW are chemical shifts of N-alkylated pyrrolic β-H corresponding to free host H and host complexed to water H · W , respectively. β δ H and β δ HW have the same values for H A and H B protons as there is no induced asymmetry here. Hence, under the above assumptions, the binding isotherm for the chemical shift difference Δ δ = β δ A − β δ B for the N-alkylated pyrrolic β-H will have the form of equation 3. The same derivation of binding isotherm applied to N-H pyrrolic β-H also applies to hemiquinonoid ortho -H resonances in case of guest 4 . How to cite this article: Labuta, J. et al . NMR spectroscopic detection of chirality and enantiopurity in referenced systems without formation of diastereomers. Nat. Commun. 4:2188 doi: 10.1038/ncomms3188 (2013).